All-back-contact ultra-thin silicon nanocone solar cells with 13.7% power conversion efficiency Thinner Si solar cells with higher efficiency can make a Si photovoltaic system a cost-effective energy solution, and nanostructuring has been suggested as a promising method to make thin Si an effective absorber. However, thin Si solar cells with nanostructures are not efficient because of severe Auger recombination and increased surface area, normally yielding <50% EQE with short-wavelength light. Here we demonstrate >80% EQEs at wavelengths from 400 to 800 nm in a sub-10-μm-thick Si solar cell, resulting in 13.7% power conversion efficiency. This significant improvement was achieved with an all-back-contact design preventing Auger recombination and with a nanocone structure having less surface area than any other nanostructures for solar cells. The device design principles presented here balance the photonic and electronic effects together and are an important step to realizing highly efficient, thin Si and other types of thin solar cells. Nanostructured solar cells have recently been investigated intensively because of their promise for low-cost materials and processing [1] , [2] , [3] , [4] , [5] , [6] , effective anti-reflection and light trapping for materials saving [7] , [8] , [9] , light-weight and mechanical flexibility for low-cost installation [10] , [11] and miniaturized energy sources [12] . However, these exciting concepts thus far give power conversion efficiency lower than their bulk counterparts. In particular, a silicon (Si) solar cell is still the mainstream technology in industry, and it has witnessed significant cost reduction in the past decade: its module cost was dropped from $33.44/W in 1980 to under $1/W in 2012 (ref. 13 ). In order to make a photovoltaic system cost-competitive without subsidies, its module cost should be <$0.5/W (ref. 14 ). Reducing a Si absorber thickness from 200 to sub-10 μm can potentially have a large impact on reducing the module cost further and enabling light-weight installation. The conventional surface texturing with alkaline or acidic solution for sub-10-μm-thick Si substrates requires additional masking steps including photolithography [15] , and it is hard to implement on thin substrates with high yield [16] . In the past several years, significant effort has been focused on enhancing the light absorption by nanoscale light trapping using nanowires [8] , [17] , [18] , [19] , nanocones [20] , [21] , [22] , nanodomes [7] and nanoholes [23] , [24] , [25] , [26] . Despite the exciting success in light trapping, the power conversion efficiencies of nanostructured Si solar cells, however, remain below 19% for thick devices [26] and below 11% for thin devices [27] . Here, we present a sub-10-μm-thick Si solar cell with a 13.7% power conversion efficiency that overcomes the critical problems of nanostructured devices: Auger and surface recombination. In general, nanostructured solar cells have a highly doped emitter layer at the front, fabricated by high-temperature diffusion processes. Because the diffusion profile of the dopants is dependent on the surface morphology, a nanostructured device tends to have a much deeper junction depth with a higher concentration compared with a planar device [26] , [28] . It leads to severe Auger and surface recombination of charge carriers [29] . Another problem of nanostructured Si solar cells is the increased surface area. For example, a porous nanostructure with ~300 nm depth and 50 nm diameter has 800% more surface area than a planar structure. Considering the fact that the surface recombination becomes more critical to device performance as the absorber becomes thinner, the increased surface area in a thin Si solar cell can lead to a severe decrease of efficiency. In particular, the increased loss to Auger and surface recombination becomes worse for short-wavelength light, which is absorbed near the surface, normally yielding <50% external quantum efficiency (EQE) at 400 nm wavelength light. Owing to these problems, thin Si solar cells with nanostructures are not as efficient as they could be. Nanostructured Si solar cell with all-back-contact design We achieved high efficiency from ultra-thin, nanostructured Si solar cells by designing an emitter layer at the back of the device rather than the front, which is a so-called all-back-contact design. As shown in Fig. 1a,b , the back side of our solar cell had an interdigitated structure of highly doped p + and n + regions. Its front side consisted of nanocones, which makes this ultra-thin device completely black. Remarkably, its EQE was >80% in the spectrum of 400–800 nm wavelengths ( Fig. 1c ), which is superior to the EQE of any other nanostructured solar cells reported so far; in particular, its EQE at 400 nm wavelength was 80%, which was at least 15% higher than that of other Si nanostructured solar cells [26] and 200% higher than that of III–V nanowire solar cells [5] . The significant light absorption, realized by the nanocones at the front, and the minimal loss of charge carriers, realized by the all-back-contact design at the back, resulted in a short-circuit current density ( J SC ) of 29.0 mA cm −2 , which is 30.7% higher than the J SC of a planar device coated with an anti-reflection layer (Si 3 N 4 , 80 nm). The current density–voltage ( J – V ) characteristics of the devices were measured under air mass 1.5 illumination, and they are presented in Fig. 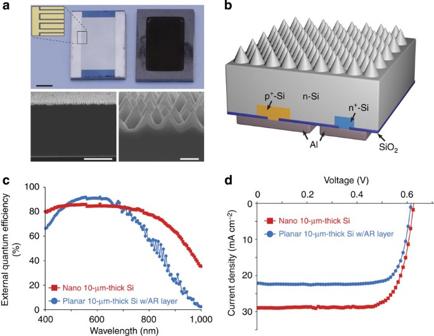Figure 1: Ultra-thin Si nanocone solar cell. (a) Optical image of the back (top, left) and front (top, right) side of the 10-μm-thick Si solar cell. Inset shows the optical microscope image of the interdigitated metal electrodes. SEM images of cross-sectional view of the device (bottom, left) and cross-sectional view of the nanocones (bottom, right). The thin layer at the top of the nanocones is an 80-nm-thick SiO2layer. Scale bars are 2 mm (top), 5 μm (bottom, left) and 400 nm (bottom, right). (b) Schematic illustration of the device. (c) EQE data of the device and a planar control. (d)J–Vcharacteristics of two devices inc. 1d and summarized in Table 1 . Figure 1: Ultra-thin Si nanocone solar cell. ( a ) Optical image of the back (top, left) and front (top, right) side of the 10-μm-thick Si solar cell. Inset shows the optical microscope image of the interdigitated metal electrodes. SEM images of cross-sectional view of the device (bottom, left) and cross-sectional view of the nanocones (bottom, right). The thin layer at the top of the nanocones is an 80-nm-thick SiO 2 layer. Scale bars are 2 mm (top), 5 μm (bottom, left) and 400 nm (bottom, right). ( b ) Schematic illustration of the device. ( c ) EQE data of the device and a planar control. ( d ) J – V characteristics of two devices in c . Full size image Table 1 Photovoltaic properties of ultra-thin Si solar cells of Fig. 1. Full size table The all-back-contact design has been used to improve the power conversion efficiency in thick Si solar cells [30] , [31] , but we found that its benefits become more significant in nanostructured thin solar cells: microstructured thick Si solar cells showed >85% EQE over the wavelengths of visible light, whether they had front–back-contact design [32] or all-back-contact design [33] . The highest power conversion efficiency of thick Si solar cells in the world was achieved with the front–back-contact design [34] . In nanostructured thin Si solar cells, however, the front–back-contact design is not effective to collect charge carriers compared with the all-back-contact design: the deeper junction depth, heavy doping at the front surface and increased surface area in a nanostructured thin solar cell lead to a severe loss of the charge carriers generated near the front ( Fig. 2a ). Considering the fact that >95% of light with 300–500 nm wavelengths is absorbed within 2 μm of the nanostructured Si surface [21] , this loss can be significant. We confirmed the benefits of the all-back-contact design in nanostructured thin solar cells using simulation. We used a TCAD (technology-computer-aided design) simulation tool, Sentaurus: the optical properties were computed using the finite-difference time-domain method and they were integrated with the device simulation. 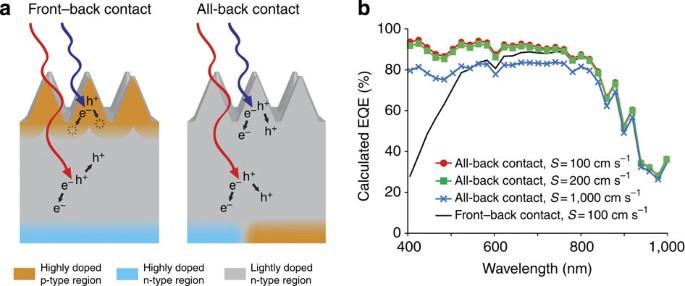Figure 2: Comparison of front–back-contact and all-back-contact designs. (a) Schematics of two different contact designs for thin Si solar cells. (b) Calculated EQE data of four different 10-μm-thick devices with the front–back-contact design and with the all-back-contact design. Figure 2b shows the calculated EQEs of four different 10-μm-thick devices. The simulation shows that the all-back-contact devices should have superior EQEs in the range of short wavelengths: with the surface recombination velocity ( S ) of 100 cm s −1 , the all-back-contact device had 94% EQE at 400 nm wavelength, whereas the front–back-contact device had only 28% EQE. The low EQE of the latter can be improved by decreasing the doping concentration at the front, but it can result in the higher series resistance and the lower efficiency. On the other hand, both devices showed similar EQEs over the spectrum of long wavelengths because light with those wavelengths is absorbed throughout the device, where the doping concentration is much lower (3 × 10 15 cm −3 ) than in the front (4 × 10 20 cm −3 ). Figure 2: Comparison of front–back-contact and all-back-contact designs. ( a ) Schematics of two different contact designs for thin Si solar cells. ( b ) Calculated EQE data of four different 10-μm-thick devices with the front–back-contact design and with the all-back-contact design. Full size image The simulation in Fig. 2b shows the importance of the surface passivation in the all-back-contact design. As the surface recombination velocity ( S ) increased from 100 to 1,000 cm s −1 , the EQE of the all-back-contact devices decreased by ~10%. This study indicates that the high EQE of our device can be increased even further by improving the passivation on its front surface. Advantages of nanocones Another reason why our nanocone solar cell demonstrates superior EQE is the minimal increase of surface area. As mentioned before, the increased surface area in a nanostructured solar cell can lead to a severe decrease of efficiency. Nanostructures for thin Si solar cells should be designed to minimize the increase in surface area while enhancing the light absorption. Our nanocone structure with a height of about 400 nm and a diameter of 450 nm ( Fig. 1b ) satisfied both requirements. The total surface area of our nanocone structure is lower than that of other nanostructured Si solar cells: it is only 67% larger than that of a planar structure, whereas the surface area of nanopores, as mentioned above, is >800% larger [26] , and that of nanowires with 4 μm height and 400 nm diameter is 2,000% larger [18] . With the smallest surface area, our nanocone structure increased the light absorption significantly: the absorption of short-wavelength light (400 nm) was 96.1%, which was 28% higher than that of the planar device coated with a 80-nm-thick Si 3 N 4 anti-reflection layer, and the absorption of long-wavelength light (900 nm) was 83.8%, which was 198% higher ( Fig. 3 ). The remarkable enhancement of light absorption in our device was achieved by the optimal balance of anti-reflection and light-scattering effects from the nanocones: we previously found that the nanocone structure with an aspect ratio (height/diameter) close to 1 is the optimal design for the light absorption in thin Si (ref. 22 ), and our nanocone had an aspect ratio of 0.9. The light absorption of our 10-μm-thick nanocone solar cell was comparable to that of 500-μm-thick planar Si coated with the anti-reflection layer (80-nm-thick Si 3 N 4 ). It should be noted that there could be some parasitic light absorption at the metal contacts. Recently, the parasitic light absorption at the back contacts becomes increasingly important because a thinner absorber layer allows more light to reach at the back of a solar cell [35] , [36] , [37] . The simulation in Fig. 4 indicates that the absorption of long-wavelength light (900 nm) at the back contacts, aluminium (Al), could increase up to 10% and 25% with and without a SiO 2 layer between Si and Al, respectively. The lower parasitic absorption with the SiO 2 layer can be due to the higher internal reflection from the back [37] . Because 60% of the back surface of our solar cell was covered with an 80-nm-thick SiO 2 layer (details in the Methods section), the parasitic absorption of long-wavelength light could be >10%. A further optimization of the back contact design will be able to increase the Si light absorption and enhance the J SC . From the light absorption measurement shown in Fig. 3 , we realized that our ultra-thin nanocone Si solar cell could achieve >34 mA cm −2 J SC . Considering the measured J SC (29 mA cm −2 ) from our device, ~5 mA cm −2 was lost because of the recombination and the parasitic absorption. 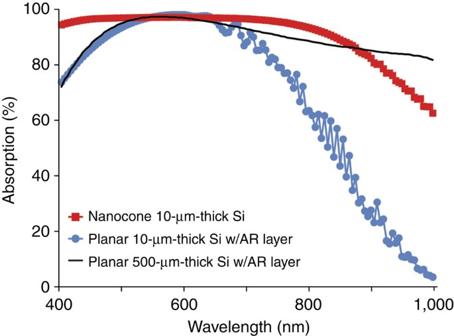Figure 3: Light absorption data of three devices. The anti-reflection (AR) layer was Si3N4with a thickness of 80 nm. Figure 3: Light absorption data of three devices. The anti-reflection (AR) layer was Si 3 N 4 with a thickness of 80 nm. 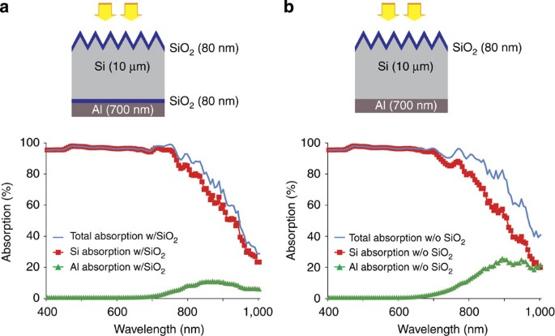Figure 4: Simulation schematics and data of light absorption in 10-μm-thick Si nanocone solar cells. (a) With a SiO2layer between Si and Al contacts. (b) Without a SiO2layer between Si and Al contacts. In order to minimize the interference pattern, the moving-average method (four-point) was applied in the data. Full size image Figure 4: Simulation schematics and data of light absorption in 10-μm-thick Si nanocone solar cells. ( a ) With a SiO 2 layer between Si and Al contacts. ( b ) Without a SiO 2 layer between Si and Al contacts. In order to minimize the interference pattern, the moving-average method (four-point) was applied in the data. Full size image Over the wavelength range of 500–700 nm, the nanocone device and the planar device absorbed similar amount of light, because the anti-reflection layer in the planar device improved the light absorption. The planar device had a smaller surface area than the nanocone device, which allowed the planar device to have lower surface recombination and higher EQEs than the nanocone device over 500–700 nm wavelengths ( Fig. 1c ). Effect of pitch between two contacts on thin Si solar cells We further exploited the advantages of the all-back-contact design in our nanostructured solar cell by optimizing the pitch between the two contacts. For thick Si solar cells with the all-back-contact design, the pitch is normally >400 μm, which allows less complicated fabrication processes such as screen-printing of metal contacts [38] , [39] , [40] . Previous studies have found that the fill factor (FF) was the only parameter that depended on the pitch in thick Si solar cells [41] , [42] . We, however, found that the J SC as well as the FF was closely dependent on the pitch in thin Si solar cells. 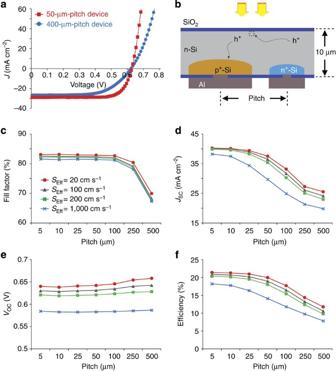Figure 5: Photovoltaic properties of 10-μm-thick Si solar cells. (a) Experimental results of 10-μm-thick Si solar cells with the same nanostructures but different pitches of the back contacts: one with 50-μm-pitch and the other with 400-μm-pitch. They are the average value from eight devices in both cases. (b) Schematic illustration of the simulated device structure. (c–f) Simulation data of FF (c),JSC(d),VOC(e) and efficiency (f) as functions of pitch and effective surface recombination velocity (SEff). Figure 5a shows the J – V characteristics of 10-μm-thick Si solar cells fabricated with the same nanostructures but different pitches between the back contacts. The FF and the J SC were increased by 23.5% and 5.4%, respectively, as the pitch decreased from 400–50 μm. The main factor for the increased FF is the decreased series resistance, R S ( Table 2 ). We used device simulation to understand these experimental results. In the simulation, we assumed no reflection from the device in order to imitate the case where there were nanocones. Figure 5b–e shows the simulation structure and data of 10-μm-thick Si solar cells as a function of the pitch. Decreases in FF and J SC with the larger pitch ( Fig. 5c,d ) can be explained by the path length over which charge carriers must diffuse to be collected in a thin device: the path length increases with the larger pitch, which results in higher series resistance and higher recombination of charge carriers, as illustrated in Fig. 5b . Because the minority carrier lifetime was 1 ms in this simulation, the recombination loss was mainly due to the surface recombination, and we confirmed that the decrease in J SC became significant as the effective surface recombination velocity ( S Eff ) increased ( Fig. 5d ). S Eff is the local surface recombination velocity ( S ) multiplied by the increased surface area: a planar device has S Eff , equivalent to S , and a nanostructured device with a N times larger surface area (compared with the planar one) has S Eff , N times larger than S [26] . Interestingly, the decrease in J SC in the experiment was much smaller than that in the simulation. It might be due to the geometric difference between the experiment (nanocone structure) and the simulation (planar structure), but the quantitative analysis on the loss mechanism of charge carriers in nanostructured and planar devices needs to be investigated further. On the other hand, the open-circuit voltage ( V OC ) increased slightly as the pitch increased, and it might be due to the decreased junction area: When the pitch was 50 μm, the n + /p + regions were 30 and 46 μm, respectively. When the pitch was 5 μm, the n + /p + regions were 3 and 4.6 μm, respectively. The pn junction area in the larger pitch device was smaller than that in the smaller pitch device, which could decrease the saturation current density and increase the V OC in the larger pitch device. However, as the S Eff increased, the effect of the junction area decreased, and the V OC became less sensitive to the pitch. These combined effects of FF, J SC and V OC indicate that nanostructured thin Si solar cells with the all-back-contact design should be designed to have both smaller pitch and less surface area. We also confirmed that the design principle, smaller pitch and less surface area, should be applied to thick solar cells, as well as thin ones, with the all-back-contact design ( Supplementary Fig. S1 ). Figure 5: Photovoltaic properties of 10-μm-thick Si solar cells. ( a ) Experimental results of 10-μm-thick Si solar cells with the same nanostructures but different pitches of the back contacts: one with 50-μm-pitch and the other with 400-μm-pitch. They are the average value from eight devices in both cases. ( b ) Schematic illustration of the simulated device structure. ( c – f ) Simulation data of FF ( c ), J SC ( d ), V OC ( e ) and efficiency ( f ) as functions of pitch and effective surface recombination velocity ( S Eff ). Full size image Table 2 Photovoltaic properties of ultra-thin Si solar cells in Fig. 5. Full size table Effect of minority carrier lifetime on thin Si solar cells Our ultra-thin Si nanocone solar cell can be fabricated with inexpensive, less-pure material. Conventional Si solar cells with the all-back-contact design need a very long lifetime of minority carriers (more than 1 ms), because their thickness is normally >150 μm and the charge carriers should diffuse to the back without recombination. This requires high-purity material and increases the solar cell cost. Our device is >15 times thinner than the conventional one, thus the charge carriers in our device need to diffuse 15 times shorter. It implies that the ultra-thin Si solar cell with the all-back-contact design can be fabricated with a less-pure material. We confirmed this benefit of the ultra-thin device using device simulation. The simulation structure was the same as shown in Fig. 5b , and the pitch was set to 50 μm. 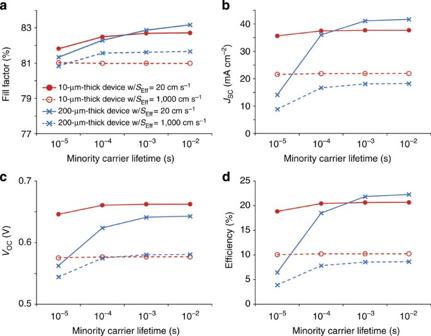Figure 6: Photovoltaic properties of thin and thick Si solar cells. Simulation data of FF (a),JSC(b),VOC(c) and efficiency (d) as functions of minority carrier lifetime and effective surface recombination velocity (SEff). Figure 6 compares the photovoltaic properties of 10- and 200-μm-thick solar cells with different minority carrier lifetimes and surface recombination velocities. With the surface recombination velocity of 20 cm s −1 , the 10-μm-thick device showed >20% efficiency as the lifetime decreased by two orders of magnitude, from 10 ms to 100 μs. When the lifetime went down to 10 μs, the efficiency was still close to 20%. In contrast, the efficiency of the 200-μm-thick device was changed significantly, from 21.8% to 6.5%, as the lifetime decreased from 1 ms to 10 μs. Interestingly, the V OC of the 10-μm-thick solar cell was higher than that of the 200-μm-thick solar cell when the S Eff was 20 cm s −1 . Because of the 20 times thinner substrate, the charge carrier concentration in the 10-μm-thick device was much higher than that of the 200-μm-thick device, which led to higher V OC [41] , [43] . This simulation study shows that well-passivated thin Si solar cells made of inexpensive material can achieve the high efficiency comparable to that of conventional thick Si solar cells made of expensive material. Figure 6: Photovoltaic properties of thin and thick Si solar cells. Simulation data of FF ( a ), J SC ( b ), V OC ( c ) and efficiency ( d ) as functions of minority carrier lifetime and effective surface recombination velocity ( S Eff ). Full size image We achieved 13.7% power conversion efficiency from a sub-10-μm-thick Si solar cell. Our ultra-thin device demonstrated more than 80% EQE at short-wavelength light, which was superior to that of any other nanostructured Si solar cell. This improvement was achieved by overcoming critical problems in nanostructured solar cells. Our device had two main advantages: the all-back-contact design and the nanocones. Its all-back-contact design prevented Auger recombination loss near the front, and its nanocone structure minimized the increase in surface area while enhancing the light absorption significantly. From the device simulation, we inferred that the effective surface recombination velocity of our ultra-thin Si solar cell was ~1000, cm s −1 and its efficiency could be higher than 20% with good surface passivation. The design principles that we outlined for highly efficient, ultra-thin Si solar cells show the potential of the nanostructured Si solar cell to be a cost-effective solution for next-generation photovoltaic devices. Si solar cell fabrication We used a silicon-on-insulator (SOI) wafer for the solar cell fabrication. Its device layer was Czochralski (CZ) Si, 10-μm thick and N-type with a resistivity of 1–5 Ω.cm. First, as a doping mask, a 300-nm-thick SiO 2 layer was grown thermally on the SOI wafer. At the surface of the device layer, interdigitated patterns for n + /p + regions were fabricated with photolithography. The widths of the n + /p + regions were 30/46 μm, respectively, and the centre-to-centre distance (pitch) between the n + and p + regions was 50 μm. After the patterning, gas-phase doping processes (n + with POCl 3 and p + with BBr 3 ) were conducted using the atmospheric furnace, tylan. The sheet resistance for the n + region was 85–90 Ω per square, and that for the p + region was 72–75 Ω per square. After the doping processes, the window patterns were defined at the back side (handle layer) of the SOI wafer: (1) the front side (device layer) was coated with 3-μm-thick photoresist for protection, (2) the SOI wafer was flip-over and (3) the back side of the SOI wafer was aligned and exposed in the ultra-violet light (365 nm). The window patterns at the back side of the wafer were etched by deep reactive-ion etching (RIE) method, which defined the solar cell area. The exposed buried oxide part was removed by wet etching, and an array of Si nanocones was fabricated by dry etching. In order to remove the surface defects formed during the nanocone fabrication process, an 80-nm-thick SiO 2 layer was grown thermally over the whole structure. The patterns for metal contacts were fabricated with photolithography at the n + /p + regions at the device layer: the widths of the contacts to the n + /p + regions were 15/25 μm, respectively. For the contacts, Al (a thickness of 700 nm) was deposited by electron-beam evaporation. Si nanocone fabrication We used colloidal lithography to make Si nanocones: (1) a monolayer of silica nanoparticles (a diameter of 500 nm) was formed on a Si substrate with the Langmuir–Blodgett method. The nanoparticles were synthesized with the modified Stöber process using the hydrolyses of tetraethyl orthosilicate in ethanol containing ammonia [44] . (2) The nanoparticles were etched by RIE to have a diameter of 200 nm. A gas mixture of oxygen (O 2 ) and trifluoromethane (CHF 3 ) was flowed with a rate of 6 and 85 sccm, respectively. These etched nanoparticles acted as a mask for Si etching. (3) The silica nanoparticles and the Si substrate were etched by RIE with a gas mixture of chlorine (Cl 2 ) and hydrogen bromide (HBr). Because of the selectivity, Si nanocones were formed in this step. Device simulation We used a TCAD simulation tool, Sentaurus, supported by Synopsys, Inc. In order to simulate the solar cell properties, we specified the following: Substrate was n-type, doped with phosphorous (a concentration of 3 × 10 15 cm −3 ). N + region was doped with phosphorous (concentration of 1 × 10 20 cm −3 , diffusion depth of 100 nm). P + region was doped with boron (concentration of 4 × 10 20 cm −3 , diffusion depth of 300 nm). The device geometry in the simulation was identical to the geometry of the real solar cell (30-μm-wide n + , 46-μm-wide p + and 50-μm-wide pitch). For the simulation of the photovoltaic properties as a function of pitch, the geometry was changed linearly: when the pitch increased to 100 μm, the widths of the n + /p + regions increased to 60/92 μm, respectively. Light absorption measurement The light transmission and reflection were measured with an integrating sphere (Newport, 3.3″ diameter). A tungsten lamp coupled to a monochromator was used as a light source. The sample was mounted at the centre of the integrating sphere, and it was rotated with an angle of 5°. There were only two holes in the integrating sphere: one for the light source and the other for the detector. After the reference signal was measured without any sample in the integrating sphere, our solar cell was mounted at the centre of the sphere. The collected light in the detector was a sum of the reflected and transmitted light from the sample. We calculated the absorption by the equation as follows: How to cite this article: Jeong, S. et al. All-back-contact ultra-thin silicon nanocone solar cells with 13.7% power conversion efficiency. Nat. Commun. 4:2950 doi: 10.1038/ncomms3950 (2013).